Solution-phase epitaxial growth of noble metal nanostructures on dispersible single-layer molybdenum disulfide nanosheets Compared with the conventional deposition techniques used for the epitaxial growth of metallic structures on a bulk substrate, wet-chemical synthesis based on the dispersible template offers several advantages, including relatively low cost, high throughput, and the capability to prepare metal nanostructures with controllable size and morphology. Here we demonstrate that the solution-processable two-dimensional MoS 2 nanosheet can be used to direct the epitaxial growth of Pd, Pt and Ag nanostructures at ambient conditions. These nanostructures show the major (111) and (101) orientations on the MoS 2 (001) surface. Importantly, the Pt–MoS 2 hybrid nanomaterials exhibit much higher electrocatalytic activity towards the hydrogen evolution reaction compared with the commercial Pt catalysts with the same Pt loading. We believe that nanosheet-templated epitaxial growth of nanostructures via wet-chemical reaction is a promising strategy towards the facile and high-yield production of novel functional materials. Epitaxial growth has been recognised as one of the most promising strategies towards the controlled growth of noble metal nanostructures (NSs) with preferred orientation and alignment on substrates, which may enable advances in many areas such as plasmonics [1] , nanoelectronics [2] , as well as the facet-selective catalysis [3] , [4] . Epitaxial growth also has a crucial role in the formation of metal-semiconductor heterostructures with the well-defined interfaces that are critical to electrical, optical and catalytic properties [5] , [6] , [7] . Vapour-phase deposition methods have been widely used to realise the epitaxial growth of noble metal NSs, such as thermal evaporation [8] , atomic layer deposition [4] and e-beam lithography [3] . Unfortunately, these deposition techniques suffer from the disadvantages of low throughput and high cost, arising from the requirement of ultra-high vacuum conditions and special equipment. As a result, the wet-chemical synthetic route remains an attractive alternative because of the relatively low cost, ease of implementation and versatility. For example, the epitaxial growth of noble metals has been demonstrated in the colloidal synthesis of bimetallic NSs [9] , [10] , [11] , [12] , [13] , which can be obtained at ambient conditions owing to the tolerable lattice mismatch (generally <5%) and favourable bonding energy between the metals [14] , [15] . However, despite the previous demonstration of metal-seeded epitaxial growth of semiconductors in solution [5] , [6] , [13] , [16] , the wet-chemical growth of metal NSs with preferred orientation and alignment on semiconductor NS templates has not been reported. This is because the nucleation of metallic domains on a semiconductor NS generally occurred on sites of defects or surfaces with a large curvature [7] . Therefore, novel synthetic template, possessing an atomically flat surface, is highly expected for realising the solution-phase epitaxy at mild experimental conditions. Two-dimensional (2D) semiconducting nanomaterials, such as graphene [17] , [18] , [19] , [20] and metal chalcogenide nanosheets [21] , [22] , have recently attracted tremendous research interest, because of their unique properties and various applications in electronics, catalysis, energy storage devices and so on. These 2D nanomaterials are also novel templates for synthesis of functional composites [17] , [23] , [24] , [25] . Recently, for the first time, we have demonstrated that graphene oxide (GO) sheets can absorb long-chain amine molecules to assist in the formation of pure hexagonal-close-packed Au nanosheets [24] . In addition, we have shown that the long-chain thiol molecules can self-assemble on the surface of reduced GO (rGO) to direct the formation of orderly aligned Au nanodot-chains [23] . However, despite the previous efforts, the epitaxial growth of noble metals on GO or rGO-based templates has not been achieved. One of the possible reasons for this is that the oxygen-containing groups on GO and rGO templates disrupt the graphitic lattice and act as nucleation sites for growth of metallic domains. However, the highly ordered pyrolytic graphite substrate, which contains much fewer surface defects as compared with GO and rGO, can facilitate the fusion of thiol-capped Ag nanoparticles (NPs) into epitaxially aligned Ag nanoplates through long time annealing (8 days) at 50 °C (ref. 26 ). Recently, we have developed an electrochemical method for facile preparation of high-yield, large-amount, single-layer metal dichalcogenide nanosheets with solution-phase processablility [27] . The obtained single-layer transition metal disulphide nanosheets, with the unique structure of transition metal atoms sandwiched inbetween two layers of hexagonally packed sulphur atoms, are potential synthetic templates for in situ growth of noble metal NSs, which have not been explored. In this contribution, we report the in situ growth of noble metal NSs (for example, Pt, Pd, Au and Ag) on single-layer molybdenum disulphide (MoS 2 ) nanosheets via wet-chemical synthesis. For the first time, the epitaxial growth of Pd, Pt and Ag NPs on MoS 2 nanosheets has been realised at ambient conditions. Two types of epitaxial orientations, that is, the (111) and (101) orientations, have been found to coexist for most metal NPs. In addition, we demonstrate that the anisotropic NS, for example, (111)-oriented triangular Ag nanoplate, can also grow and epitaxially align on the MoS 2 nanosheets. Importantly, the Pt–MoS 2 hybrid nanomaterials have been used as promising catalysts for the hydrogen evolution reaction (HER), which exhibited much better electrocatalytic activity compared with the commercial Pt catalyst at the same Pt loading. Our results indicate that the solution synthesis of noble metal NSs with preferred orientation and alignment on the dispersible semiconductor nanosheets provides a new strategy for the facile and high-yield preparation of novel functional materials. Epitaxial growth of Pd, Pt and Ag NSs on MoS 2 nanosheets After the single-layer MoS 2 nanosheets in water were prepared using our recently developed method [27] (confirmed by the AFM measurement shown in Supplementary Fig. S1 ), the noble metal NSs were synthesised in situ on the MoS 2 surface. Depending on the different metal precursors used, that is, K 2 PtCl 4 , K 2 PdCl 4 , HAuCl 4 or AgNO 3 , different reduction methods were applied, such as chemical reduction with ascorbic acid or NaBH 4 , the photochemical reduction or the electroless deposition (see the detailed synthetic methods in the Methods section). For example, Pd NPs were synthesised on MoS 2 nanosheets by reduction of K 2 PdCl 4 with ascorbic acid in the presence of cetyltrimethylammonium bromide (CTAB). As shown in the transmission electron microscopy (TEM) image in Fig. 1a , Pd NPs with size of ~5 nm were adsorbed on the surface of the MoS 2 nanosheet. Detailed TEM analysis was then carried out on these Pd–MoS 2 hybrid nanomaterials ( Fig. 1b–d and Supplementary Fig. S2a ), which clearly demonstrated the epitaxial growth of Pd NPs on the MoS 2 surface. As shown in Fig. 1b , the selected area electron diffraction (SAED) pattern of a Pd–MoS 2 hybrid nanomaterial, with the basal plane of MoS 2 nanosheet normal to the electron beam, gives two sets of diffraction spots, assigned to MoS 2 and Pd, respectively. The six spots of {202} Pd planes, with a corresponding lattice spacing of ~1.4 Å, are aligned with the six spots of {110} MoS2 with a lattice spacing of ~1.6 Å. Besides, another six spots of Pd, which are aligned with the six spots of {100} MoS2 , show a corresponding lattice spacing of 2.2–2.4 Å ( Supplementary Fig. S3a ). These six spots of Pd can be assigned to both the {111} Pd and 1/3{422} Pd planes with theoretical lattice spacings of 2.21 and 2.35 Å, respectively. Note that the diffraction spots for {111} Pd and 1/3{422} Pd planes are too close to be distinguished in the SAED pattern. As the orientation of the synthesised Pd NPs cannot be confirmed only by the SAED pattern, high-resolution TEM (HRTEM) characterisation was carried out ( Fig. 1c ). The measured lattice spacing of 2.7 Å with six-fold symmetry can be assigned to the {100} planes of the MoS 2 nanosheet. The fast Fourier transfer (FFT) generated SAED patterns of the Pd NPs in Fig. 1c were shown in Supplementary Fig. S3d–h to indicate their orientations. After investigation of more than 50 Pd NPs, we found that the majority (~70%) of them lie on the MoS 2 nanosheets with either the (111) Pd or (101) Pd orientation. Note that ±10° angular misorientation was allowed during the counting of the epitaxial NPs. For the (101)-oriented Pd NPs, the lattice fringes with inter-plane spacings of 2.2 and 1.9 Å were clearly observed, which can be attributed to the {111} Pd and {200} Pd planes, respectively ( Fig. 1c ). In addition, the direction of a (101)-oriented Pd NP is aligned with one of the six equivalent <100> directions of MoS 2 . For the (111)-oriented Pd NPs, on the other hand, the lattice spacing of ~2.4 Å with hexagonal lattice patterning can be assigned to the 1/3{422} Pd planes. The presence of the forbidden diffraction spots of 1/3{422} planes can be attributed to several possible reasons, such as the small thickness of the crystal with an atomic layer number that is not an integral multiple of 3, or the presence of stacking faults parallel to the (111) basal plane [28] . Occasionally, the (111)-oriented Pd NP with {220} Pd lattice spacing of ~1.4 Å can also be observed ( Fig. 2d ). For these (111)-oriented Pd NPs, their <110> directions are aligned with the six equivalent <100> directions of MoS 2 . These observations are in agreement with the lattice relationship indicated by the SAED pattern in Fig. 1b . Besides these two types of oriented Pd NPs, the randomly oriented NPs were also observed, which led to the weak and discontinuous diffraction rings of Pd{111}, {200} and {220} planes in the SAED pattern ( Fig. 1b ). This may arise from the random nucleation of Pd NPs on the surface defects of MoS 2 ( Supplementary Fig. S4 ). Based on the SAED and HRTEM data, two types of epitaxial relationship between the Pd NPs and MoS 2 nanosheet were confirmed and defined by (1) Pd || [100] MoS2 and (101) Pd || (001) MoS2 and (2) Pd || [100] MoS2 and (111) Pd || (001) MoS2 , respectively. 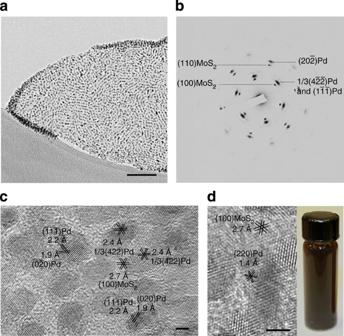Figure 1: TEM analysis of Pd–MoS2hybrid nanomaterials. (a) TEM image of Pd NPs synthesised on an MoS2nanosheet (scale bar, 50 nm). (b) SAED pattern of a Pd–MoS2hybrid nanosheet with the electron beam perpendicular to the basal plane of the MoS2nanosheet. (c,d) HRTEM images of Pd NPs on MoS2, showing distinguishable lattice fringes for Pd and MoS2(scale bar, 2 nm). Inset in (d): photograph of the Pd–MoS2solution. Figure 1: TEM analysis of Pd–MoS 2 hybrid nanomaterials. ( a ) TEM image of Pd NPs synthesised on an MoS 2 nanosheet (scale bar, 50 nm). ( b ) SAED pattern of a Pd–MoS 2 hybrid nanosheet with the electron beam perpendicular to the basal plane of the MoS 2 nanosheet. ( c , d ) HRTEM images of Pd NPs on MoS 2 , showing distinguishable lattice fringes for Pd and MoS 2 (scale bar, 2 nm). Inset in ( d ): photograph of the Pd–MoS 2 solution. 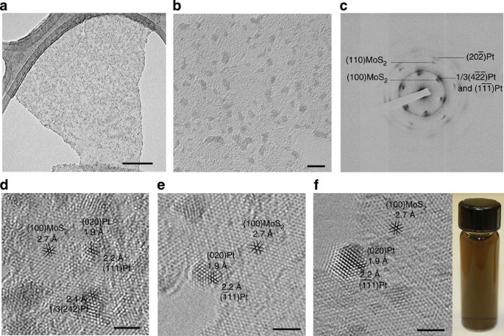Figure 2: TEM analysis of Pt–MoS2hybrid nanomaterials. (a) TEM image of Pt NPs synthesised on an MoS2nanosheet (scale bar, 100 nm). (b) Magnified TEM image of Pt NPs on MoS2nanosheet. The size of the Pt NPs is 1–3 nm (scale bar, 5 nm). (c) SAED pattern of a Pt–MoS2hybrid nanosheet with the electron beam perpendicular to the basal plane of the MoS2nanosheet. (d–f) HRTEM image of Pt NPs on MoS2showing distinguishable lattice fringes for Pt and MoS2(scale bar, 2 nm). Inset in (f): photograph of the Pt–MoS2solution. Full size image Figure 2: TEM analysis of Pt–MoS 2 hybrid nanomaterials. ( a ) TEM image of Pt NPs synthesised on an MoS 2 nanosheet (scale bar, 100 nm). ( b ) Magnified TEM image of Pt NPs on MoS 2 nanosheet. The size of the Pt NPs is 1–3 nm (scale bar, 5 nm). ( c ) SAED pattern of a Pt–MoS 2 hybrid nanosheet with the electron beam perpendicular to the basal plane of the MoS 2 nanosheet. ( d – f ) HRTEM image of Pt NPs on MoS 2 showing distinguishable lattice fringes for Pt and MoS 2 (scale bar, 2 nm). Inset in ( f ): photograph of the Pt–MoS 2 solution. Full size image To form the Pt–MoS 2 hybrid nanomaterials, an in situ photochemical reduction route was applied (see the Methods section for the detailed experiment). Similar with the Pd NPs, most of the 1–3 nm Pt NPs also epitaxially grew on the MoS 2 nanosheet ( Fig. 2 and Supplementary Fig. S2b ). As indicated by the SAED pattern of a Pt–MoS 2 hybrid nanomaterial ( Fig. 2c ), the {111} (or 1/3{422}) and {202} spots of Pt are evidently aligned with the {100} and {110} diffraction spots of MoS 2 , respectively. However, because of the smaller size of the Pt NPs compared with the Pd NPs, the diffraction spots of Pt are relatively weak. The continuous diffraction rings of {111}, {200} and {220} of Pt were also identified, suggesting that a portion of the synthesised Pt NPs (~35% of surveyed Pt NPs) did not epitaxially grow on MoS 2 . The HRTEM image of Pt NPs on MoS 2 ( Fig. 2d and Supplementary Fig. S5 ) shows that most Pt NPs are oriented along either the [101] or [111] zone axis, with their or directions aligned with one of the <100> directions of MoS 2 , respectively. Therefore, similar with the Pd–MoS 2 hybrid materials, two types of epitaxial relationship between the Pt NPs and MoS 2 nanosheets can be defined by (1) Pt || [100] MoS2 and (101) Pt || (001) MoS2 and (2) Pt || [100] MoS2 and (111) Pt || (001) MoS2 , respectively. Furthermore, the epitaxial growth of Ag NPs on MoS 2 has also been realised (see Supplementary Fig. S6 and the description in the Methods section). In contrast to Pt, Pd and Ag, the reduction of HAuCl 4 in the presence of MoS 2 was spontaneous without the addition of any reducing agent. Such electroless deposition of metal on substrate has also been observed previously in the syntheses of Ag on Si or Ge [29] , Au on a single wall carbon nanotube [30] and Ag on graphene [31] . Because of the rapid reduction and formation of dendritic Au NSs with high-density defects, the epitaxial growth was not observed in the Au–MoS 2 hybrid materials ( Supplementary Fig. S7 ). On the basis of the aforementioned observation and analyses, the crystal models for epitaxial growth of Pd, Pt and Ag on MoS 2 nanosheets are schematically illustrated in Fig. 3a for the (111) and (101) orientations, respectively. Note that Li-intercalated and exfoliated MoS 2 nanosheets are composed of 2H and 1T polymorphs [32] , proved by the deconvolution of X-ray photoelectron spectroscopy (XPS) Mo3d bands ( Supplementary Fig. S8 ). The 2H and 1T structures are different in the stacking order of S-Mo-S sandwiched tri-layer, that is, the stacking order of S-Mo-S in the 2H structure is a-B-a and that in the 1T structure is a-B-c ( Supplementary Fig. S9 ). The sulphur layers in both the 2H and 1T structures are hexagonal-close-packed with the same surface atomic structure [33] . As the deposited metal NPs are attached to the S layer, their epitaxial relationship to the 2H or 1T structure can be illustrated using the same model ( Fig. 3 ). The lattice constants for the noble metals with face-centered cubic structure are: a Pt =3.92 Å (ICSD no. 76153), a Pd =3.89 Å (ICSD no. 76148) and a Ag =4.09 Å (ICSD no. 64706); and those for 2H-MoS 2 are: a =3.16 and c =12.30 (ICSD no. 84180). Therefore, in the case of the (111) orientation, the calculated lattice mismatch along the M || [100] MoS2 direction is about 12%, 13% and 9% for Pt, Pd and Ag, respectively. The (111) orientation has also been previously demonstrated in the vapour-phase deposition of noble metals on the cleaved MoS 2 substrate [34] . However, the second type of epitaxy, that is, the (101) orientation ( Fig. 3b ), was unexpected, because the metal (101) plane and MoS 2 (001) plane are different in crystalline symmetry, accompanied with a large lattice mismatch. 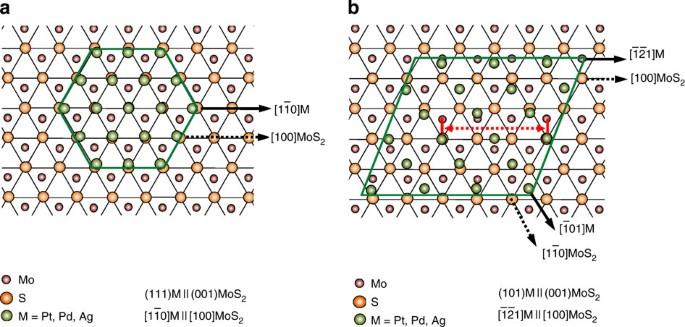Figure 3: Schematic illustration of the epitaxial growth of metal NPs on MoS2. Azimuthal orientation of a metal NP on the MoS2(001) surface in the (a) (111) and (b) (101) orientations. Only the first S layer and the second Mo layer are drawn in the scheme. Figure 3: Schematic illustration of the epitaxial growth of metal NPs on MoS 2 . Azimuthal orientation of a metal NP on the MoS 2 (001) surface in the ( a ) (111) and ( b ) (101) orientations. Only the first S layer and the second Mo layer are drawn in the scheme. Full size image In order to justify the observed epitaxial growth of the (101)-oriented Pd, Pt and Ag NPs on MoS 2 sheets, we applied the model of domain-matching epitaxy [35] , [36] , [37] , in which the lattices of substrate and overlayer match through a domain that contains integral numbers of lattice layers. Taking Pd as an example, the lattice mismatch of a (101)-oriented Pd NP on (001) MoS2 is 13.0% along the pd direction with a 5 o of angular misorientation (with respect to the MoS2 direction), and 50.6% along the Pd direction. However, if we consider a domain containing two layers of Pd atoms and three layers of S atoms in MoS 2 , the mismatch along the Pd direction becomes only 0.4% (indicated by the red arrow in Fig. 3b ), which makes it possible to grow the (101)-oriented NPs on MoS 2 . The same model has also been applied previously to explain the growth of (101)-oriented Au, Pd and Au/Pd nanowires on c-cut sapphire via the chemical vapour deposition [8] . To further demonstrate the general applicability of the solution-phase epitaxy of nobel metals on dispersible 2D nanomaterials, we have grown the anisotropic metal NSs, that is, the (111)-oriented Ag nanoplates, with well-defined shape and surface alignment, on MoS 2 . Here we used a modified synthetic procedure to prepare the Ag nanoplates, where AgNO 3 was reduced by NaBH 4 in the presence of polyvinylpyrrolidone (PVP), trisodium citrate and H 2 O 2 (ref. 38 ). In this approach, H 2 O 2 is an important reactant. During the early stage of particle growth, it etches away the unstable NPs with defects and leaves the most stable ones, that is, the nanoplates, enclosed by two parallel {111} basal planes [39] . As shown in Fig. 4a , Ag nanoplates with edge length of 30–60 nm were synthesised on the MoS 2 nanosheet. In Fig. 4a , three dashed lines indicate that 80% of the nanoplates are aligned on the MoS 2 nanosheet. The detailed TEM analysis was then carried out on a typical Ag nanoplate ( Fig. 4b–d ). The FFT-SAED pattern of Fig. 4d indicates that the 1/3{422} plane of the Ag nanoplate is aligned with the {100}MoS 2 plane with an angular misorientation of ~6° ( Fig. 4c ). The filtered HRTEM image obtained by selecting the diffraction spots of Ag shows a lattice spacing of 2.5 Å, assigned to the 1/3{422} Ag planes ( Fig. 4d ). The SAED pattern of several Ag nanoplates on MoS 2 further illustrates the 1/3{422} Ag ||{100} MoS2 epitaxial relationship ( Supplementary Fig. S10 ), although some nanoplates show an angular misorientation of 0–10°. The angular misorientation, which is larger than that of the Ag plates formed on the highly ordered pyrolytic graphite surface [16] , might arise from the surface defects of MoS 2 nanosheets ( Supplementary Fig. S4 ) and the presence of surface capping molecules [26] , as well as the vigorous decomposition of H 2 O 2 to release gaseous oxygen during the synthesis. 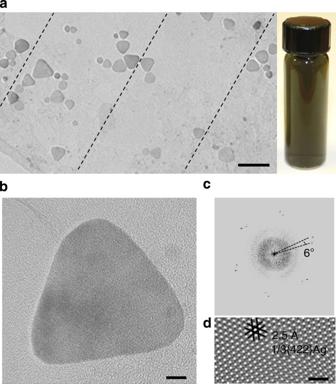Figure 4: TEM analysis of Ag–MoS2hybrid nanomaterials. (a) TEM image of Ag nanoplates synthesised on an MoS2nanosheet. Three dashed parallel lines indicate the alignment of the Ag nanoplates on substrate (scale bar, 100 nm). (b) TEM image of a typical Ag nanoplate on MoS2nanosheet (scale bar, 10 nm). (c) FFT-generated SAED pattern of (b). (d) Filtered HRTEM image of the Ag nanoplate in (b) (scale bar, 2 nm). Inset in (a): photograph of the Ag–MoS2solution. Figure 4: TEM analysis of Ag–MoS 2 hybrid nanomaterials. ( a ) TEM image of Ag nanoplates synthesised on an MoS 2 nanosheet. Three dashed parallel lines indicate the alignment of the Ag nanoplates on substrate (scale bar, 100 nm). ( b ) TEM image of a typical Ag nanoplate on MoS 2 nanosheet (scale bar, 10 nm). ( c ) FFT-generated SAED pattern of ( b ). ( d ) Filtered HRTEM image of the Ag nanoplate in ( b ) (scale bar, 2 nm). Inset in ( a ): photograph of the Ag–MoS 2 solution. Full size image Electrocatalytic activity of Pt–MoS 2 nanomaterials for HER The capability of producing functional hybrid materials in large amount at low cost is one of the most important advantages of wet-chemical synthesis. As a proof of concept, Pt NPs epitaxially grown on MoS 2 were used as a hybrid catalyst for the HER. In order to compare the electrocatalytic activity between Pt–MoS 2 hybrid materials (36 wt% Pt in Pt–MoS 2 , Supplementary Fig. S11 ) and the commercial hydrogenation Pt catalyst (10% Pt on activated charcoal, referred to as Pt–C, with Pt particle size of 1–3 nm as shown in Supplementary Fig. S12 ), we tested these two catalysts on the basis of equal Pt loading. As shown in Fig. 5a , both the synthesised Pt–MoS 2 and commercial Pt–C catalysts exhibit excellent electrocatalytical activities towards HER with negligible overpotentials. Importantly, at the same potential, the Pt–MoS 2 catalyst afforded significantly higher current density than did the commercial Pt–C ( Fig. 5a ). As a control experiment, the HER of pure MoS 2 was also tested. However, it showed a much lower activity compared with Pt–MoS 2 and Pt–C. The calculated Tafel slopes for Pt–C, Pt–MoS 2 and MoS 2 are 30, 40 and 94 mV per decade, respectively ( Fig. 5b ). It indicates that the catalytic reaction for Pt–MoS 2 proceeds via the combination of Volmer–Tafel and Volmer–Heyrovsky mechanisms, whereas in the pure MoS 2 catalysed reaction, the Volmer reaction (or the primary discharge step) is the rate-determining step [40] , [41] . Therefore, despite the 64 wt% content of MoS 2 in the Pt–MoS 2 hybrid nanomaterials ( Supplementary Fig. S11 ), Pt NPs contributed mostly to the electrocatalytic HER current. 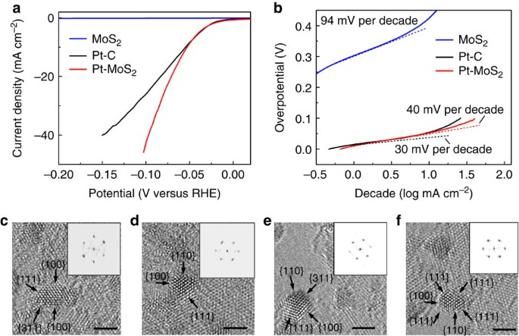Figure 5: Electrocatalytic activity of Pt–MoS2hybrid nanomaterials for the hydrogen evolution reaction and HRTEM analysis of Pt–MoS2hybrid nanomaterials. (a) Polarisation curves obtained on rotating disk glassy carbon electrodes with a loading of 0.075 (Pt–MoS2), 0.27 (Pt–C) and 0.027 (MoS2) mg cm−2, respectively. The Pt loading (0.027 mg cm−2) kept the same for the Pt–MoS2and Pt–C electrodes. Linear sweep voltammetry with a scan rate of 2 mV s−1was conducted in 0.5 M H2SO4at an electrode rotating speed of 1,000 r.p.m. N2was purged before the measurements. (b) The corresponding Tafel plots. The dashed lines indicate the linear regions, which were used to calculate the Tafel slopes. (c–f) HRTEM images of (101)-oriented Pt NPs on MoS2(scale bar, 2 nm), revealing the exposed {110} or/and {311} facets in addition to the {100} and {111} facets, indicated by the arrowheads, which are drawn perpendicular to the exposed facets. Insets in (c–f): the FFT-generated SAED patterns of the corresponding Pt NPs shown in (a–d), indicating that they are oriented along the <101> zone axis. Figure 5: Electrocatalytic activity of Pt–MoS 2 hybrid nanomaterials for the hydrogen evolution reaction and HRTEM analysis of Pt–MoS 2 hybrid nanomaterials. ( a ) Polarisation curves obtained on rotating disk glassy carbon electrodes with a loading of 0.075 (Pt–MoS 2 ), 0.27 (Pt–C) and 0.027 (MoS 2 ) mg cm −2 , respectively. The Pt loading (0.027 mg cm −2 ) kept the same for the Pt–MoS 2 and Pt–C electrodes. Linear sweep voltammetry with a scan rate of 2 mV s −1 was conducted in 0.5 M H 2 SO 4 at an electrode rotating speed of 1,000 r.p.m. N 2 was purged before the measurements. ( b ) The corresponding Tafel plots. The dashed lines indicate the linear regions, which were used to calculate the Tafel slopes. ( c – f ) HRTEM images of (101)-oriented Pt NPs on MoS 2 (scale bar, 2 nm), revealing the exposed {110} or/and {311} facets in addition to the {100} and {111} facets, indicated by the arrowheads, which are drawn perpendicular to the exposed facets. Insets in ( c – f ): the FFT-generated SAED patterns of the corresponding Pt NPs shown in ( a – d ), indicating that they are oriented along the <101> zone axis. Full size image In order to explain the obtained good catalytic activity, we examined the exposed facets of the Pt NPs. It has been known that Pt-catalysed HER is a structure-sensitive process [42] . The HER activity on low index Pt facets in the acid media is in the order of Pt{111}<Pt{100}<Pt{110} [40] , [42] , arising from the different adsorption energies of active intermediates on different Pt facets. High index facets such as Pt{311} also provide step sites for the effective adsorption of hydrogen intermediate species, which may be important for activation of HER [43] . As shown in Supplementary Fig. S5c–f , in addition to the {111} and {100} facets, {110} and {311} facets were also observed in the Pt NPs synthesised on MoS 2 . Moreover, XPS was used to obtain the information on the oxidation states of Pt–MoS 2 hybrid nanomaterials ( Supplementary Fig. S13 ). The absence of Pt 0 and the presence of the major Pt δ+ bands likely results from the substrate-catalyst interaction, that is, the electron transfer from the Pt NPs to the MoS 2 nanosheet [44] , [45] . In addition, the 2D nanosheets provide large specific surface area and can easily collect and transport charges in a 3D matrix [46] , which are beneficial to the efficient charge transfer and ionic interchange at the catalyst surface. In the solution-phase synthesis of metal NSs, factors such as surfactant molecules and reducing agents have important roles in controlling the nucleation rate, size uniformity, crystallinity and morphology of the resulting metal NSs [47] , [48] . Therefore, besides choosing a dispersible 2D template with suitable lattice parameters to induce the epitaxial growth of metal NSs, the following experimental conditions are also required in order to realise the solution-phase epitaxial growth. First, a mild reducing environment is required, so that the metal NSs can preferably nucleate on the 2D template rather than in the solution. In our experiments, mild synthetic approaches, such as photochemical reduction, and chemical reduction with ascorbic acid, were employed. Taking the photochemical reduction of Pt as an example, it was observed that small Pt clusters firstly formed at the edge sites of the MoS 2 nanosheet after the photo-reduction process proceeded for 30 min ( Supplementary Fig. S14a ). These Pt clusters showed an inter-atomic distance R Pt-Pt of ~2.8–2.9 Å ( Supplementary Fig. S14b,c ) [49] , [50] , larger than that of face-centered cubic Pt NPs ( R pt-pt =2.77 Å with a lattice constant of a =3.92 Å, ICSD no. 76153). During the next 1.5 h of photo-reduction, we observed crystallisation of the Pt clusters and growth of more Pt NPs with sizes of 1–3 nm on the MoS 2 nanosheets ( Fig. 2 ). In contrast, in the absence of MoS 2 nanosheets, the photochemical reduction of K 2 PtCl 4 led to the formation of aggregates of large Pt NPs with sizes of ~30 nm ( Supplementary Fig. S15 ). Therefore, MoS 2 nanosheets not only provided plenty of nucleation sites for the growth of Pt NPs, but also stabilised these small NPs and prevented them from aggregation. Second, the use of surface capping agents, like sodium citrate, PVP or CTAB, is essential to control the crystallinity and uniformity of NPs. As only one side of a metal NP is in contact with the 2D epitaxial template, the growth of the NP in the other directions has to be confined or kinetically controlled by surface capping molecules. For example, some control experiments were conducted for synthesising Pd and Ag NSs on MoS 2 in the absence of CTAB or PVP. As shown in Supplementary Fig. S16a,b , without adding CTAB into the growth solution, the synthesised Pd NPs were irregularly shaped with a high density of defects. As for the preparation of Ag–MoS 2 hybrid nanomaterials, although Ag nanoplates can be synthesised on MoS 2 in the absence of PVP ( Supplementary Fig. S16c ), large amount of Ag spherical NPs and irregularly shaped Ag NSs were also observed. Third, different experimental conditions have been used to produce anisotropic metal NSs. For example, in order to synthesise Ag nanoplates, NaBH 4 was used as the reducing agent in the presence of H 2 O 2 , which can etch away the unstable Ag particles with defects and leave those stable ones with exposed (111) facets. At the same time, the MoS 2 template determined the surface alignment of the resulting Ag nanoplates. In summary, the epitaxial growth of Pd, Pt and Ag NPs on MoS 2 nanosheets has been realised via wet-chemical synthesis at ambient conditions. Two types of epitaxial orientations, that is, the (111) and (101) orientations, have been observed for most metal NPs. As for the anisotropic NSs, like triangular Ag nanoplates, the preferred (111) orientation and the epitaxial surface alignment have also been demonstrated. Importantly, the Pt–MoS 2 hybrid nanomaterial showed the better catalytic activity than did the commercial Pt catalyst for the HER at the same Pt loading. Our results demonstrate that the use of novel 2D semiconductor nanosheets as synthetic templates for the solution-phase epitaxial growth of metal NSs is a promising way towards the facile, economical and high-yield preparation of novel functional hybrid nanomaterials. Chemicals MoS 2 (10–30 μm) was purchase from Rose Mill (West Hartford, USA). Lithium ion battery electrolyte was purchased from Charslton Technologies Pte Ltd (International Business Park, Singapore). Lithium foil and copper foil were purchased from ACME Research Support Pte Ltd (Bukit Batok Street, Singapore). Acetone (Tech Grade) was purchased from Aik Moh Paints and Chemicals Pte Ltd (Singapore). Ethanol (absolute >99.9%) was purchased from Merck (Darmstadt, Germany). Polypropylene (PP) film was purchase from Celgard 2300 (North Carolina, USA). Poly (vinylidene fluoride) (PVDF), N-methylpyrrolidone, gold(III) chloride hydrate (~50% Au basis), silver nitrite (99.98% trace metals basis), potassium tetrachloroplatinate(II) (99.99% trace metals basis), potassium tetrachloropalladate(II) (99.99% trace metals basis), sodium borohydride (99.99%), hexadecyltrimethylammonium bromide, L -ascorbic acid, PVP (powder, average Mw ~29,000), platinum on activated charcoal (hydrogenation catalyst, 10% Pt basis) and sodium citrate tribasic dehydrate (ACS reagent, ≥99.0%) were purchased from Sigma-Aldrich (Steinheim, Germany). All chemicals were used as received without further purification. The deionised water was purified using Milli-Q System (Millipore, Billerica, MA, USA). Electrochemical intercalation Based on our recent work [27] , lithium intercalation of the layered materials was performed in a test cell using the Li foil as anode and 1 M LiPF 6 as electrolyte, which was dissolved in a mixture of ethyl carbonate and dimethyl carbonate with a volume ratio of 1:1. The bulk MoS 2 powder (2 mg) mixed with acetylene black and PVDF binder dispersed in N -methylpyrrolidone was used as cathode. In the mixed slurry, the mass ratio of MoS 2 , acetylene black and PVDF was 80:10:10. The resulting slurry was then uniformly coated on a copper foil and dried under vacuum overnight. The electrochemical intercalation of the layered materials in the test cell was accomplished in a Neware battery test system at room temperature. The electrochemical intercalation was performed using the galvanostatic discharge at current density of 0.05 mA. After the discharge process, the Li-intercalated sample (prepared from 2 mg MoS 2 ) was washed with acetone to remove any residual electrolyte (LiPF 6 ), followed by exfoliation and ultrasonication in 20 ml distilled water to obtain the 0.1 mg ml −1 MoS 2 solution. Synthesis of Pd–MoS 2 hybrid nanomaterials After 2 ml of 0.1 mg ml −1 MoS 2 solution was centrifuged at 8,500 r.p.m. for 20 min, the supernatant was removed and the precipitate was re-dispersed in 8 ml fresh growth solution containing 20 mM CTAB and 0.5 mM K 2 PdCl 4 in water. Into this solution, 320 μl aqueous solution of 50 mM ascorbic acid and 320 μl aqueous solution of 0.5 M NaOH were added in sequence with mild shaking. After 1 h, the resulting solution was centrifuged at 60,000 r.p.m. for 10 min, and the precipitate was re-dispersed in water before further characterisation. Synthesis of Pt–MoS 2 hybrid nanomaterials After 2 ml (or 4 ml for a less amount of Pt loading) of 0.1 mg ml −1 MoS 2 solution was centrifuged at 8,500 r.p.m. for 20 min, the supernatant was removed and the precipitate was re-dispersed in 8 ml fresh growth solution containing 0.2 mM K 2 PtCl 4 and 0.3 mM trisodium citrate in water. This mixed solution in a 10-ml glass vial was then irradiated with a 150-W halogen lamp at 80% of its full intensity for 2 h, during which the glass vial was cooled by ice water to prevent the light-induced overheating. After the reaction, the resulting solution was centrifuged at 7,500 r.p.m. for 15 min, and the precipitated Pt–MoS 2 hybrid nanomaterials were re-dispersed in 0.3 mM sodium citrate solution before further characterisation. In addition, the Pt–MoS 2 hybrid nanomaterials can also be obtained by photo-irradiation at 30% of the lamp intensity for 10 h. In this case, the ice-bath cooling is not required. Synthesis of Au–MoS 2 hybrid nanomaterials After 2 ml of 0.1 mg ml −1 MoS 2 solution was centrifuged at 8,500 r.p.m. for 20 min, the supernatant was removed and the precipitate was re-dispersed in 8 ml aqueous solution containing 0.3 mM trisodium citrate. Into this solution, 80 μl of 20 mM HAuCl 4 aqueous solution was added with mild shaking. Within 5 s, the solution colour turned from dark green to grey, indicating the reduction of HAuCl 4 . The resulting solution was then centrifuged at 6,000 r.p.m. for 10 min, and the precipitate was re-dispersed in water before further characterisation. Note that without the presence of trisodium citrate, the deposition of Au NSs on MoS 2 nanosheets can also occur. In our synthesis, the trisodium citrate served as a surface capping agent for the better dispersion of the Au–MoS 2 hydrid nanomaterials in water. Synthesis of Ag–MoS 2 hybrid nanomaterials After 2 ml of 0.1 mg ml −1 MoS 2 solution was centrifuged at 8,500 r.p.m. for 20 min, the supernatant was removed and the precipitate was re-dispersed in 8 ml aqueous solution containing 0.1 mM AgNO 3 and 20 mM CTAB. Into this solution, 64 μl aqueous solution of 50 mM ascorbic acid, 6.4 μl aqueous solution of 0.5 M NaOH and ice-water cold 50 μl aqueous solution of 100 mM NaBH 4 were added in sequence. After 10 min of reaction, the resulting solution was centrifuged at 6,000 r.p.m. for 10 min, and the obtained precipitate was re-dispersed in water before further characterisation. Synthesis of Ag nanoplate–MoS 2 hybrid nanomaterials After 2 ml of 0.1 mg ml −1 MoS 2 solution was centrifuged at 8,500 r.p.m. for 20 min, the supernatant was removed and the precipitate was re-dispersed in 100 μl water. In a 10-ml glass vial, 7.5 ml water was mixed with 80 μl aqueous solution of 10 mM AgNO 3 , 32 μl aqueous solution of PVP (5 wt%, average M w ~29,000) and 19.2 μl H 2 O 2 (30%) under vigorous stirring in the open air. Into this solution, 50 μl of 100 mM NaBH 4 cooled by ice water, and 100 μl MoS 2 solution were added in sequence while stirring. Then the vial was tightly capped and left undisturbed. In about 40 min, the solution colour changed from deep green to purple, and finally to deep blue, indicating the formation of Ag nanoplates. The resulting solution was centrifuged at 5,000 r.p.m. for 10 min, and the obtained precipitate was re-dispersed in water before further characterisation. Electrocatalytic measurements Three types of catalysts were tested for the HER, including the commercial 10 wt% Pt on activated charcoal (Pt–C), MoS 2 -Pt and MoS 2 . The dispersion of Pt–MoS 2 (or MoS 2 ) was prepared by 30-min sonication of a mixture containing 0.05 ml of 2.5 mg ml −1 MoS 2 -Pt solution (or 0.05 ml of 0.9 mg ml −1 MoS 2 nanosheet solution), 0.04 ml H 2 O, 0.023 ml ethanol. The Pt–C catalyst dispersion was prepared by 30-min sonication of a mixture containing 4 mg 10 wt% Pt on activated charcoal, 0.8 ml H 2 O, 0.2 ml ethanol. Then 4.8 μl of the catalyst dispersion (containing 19.2 μg Pt–C, 5.3 μg Pt–MoS 2 or 1.9 μg MoS 2 ) was loaded onto a glassy carbon electrode and naturally dried overnight. As the diameter of electrode is 3 mm, the loading of Pt–C, Pt–MoS 2 and MoS 2 was 0.27, 0.075 and 0.027 mg ml −1 , respectively. Note that the Pt content in the Pt–MoS 2 hybrid nanomaterials is 36 wt% ( Supplementary Fig. S8 ). Therefore, the loading of Pt is same (~0.027 mg ml −1 ) for both the Pt–C and Pt–MoS 2 electrodes. Linear sweep voltammetry with a scan rate of 2 mV s −1 was conducted in 0.5 M H 2 SO 4 using 3 M Ag/AgCl electrode as the reference electrode, a Pt wire as the counter electrode and the rotating disk glassy carbon electrode as the working electrode with a rotating speed of 1,000 r.p.m. The 3 M Ag/AgCl was used as the reference in all measurements, and all the potentials were converted to values with reference to a reversible hydrogen electrode. Cyclic voltammetries were carried out at a scan rate of 100 mV s −1 . Characterisation A drop of a solution containing the synthesised MoS 2 -templated hybrid nanomaterials was placed on a holey carbon-coated copper grid, Si/SiO 2 and glass, and then naturally dried in air before characterisation by TEM (JEM 2100F), XPS (Axis Ultra), and X-ray diffraction (Shimadzu), respectively. How to cite this article: Huang, X. et al . Solution-phase epitaxial growth of noble metal nanostructures on dispersible single-layer molybdenum disulphide nanosheets. Nat. Commun . 4:1444 doi: 10.1038/ncomms2472 (2013).